Synapse microarray identification of small molecules that enhance synaptogenesis Synaptic function is affected in many brain diseases and disorders. Technologies for large-scale synapse assays can facilitate identification of drug leads. Here we report a 'synapse microarray' technology that enables ultra-sensitive, high-throughput and quantitative screening of synaptogenesis. Our platform enables the induction of synaptic structures in regular arrays by precise positioning of non-neuronal cells expressing synaptic proteins, while allowing neurites to grow freely around these cells. The technology increases by tenfold the sensitivity of the traditional assays, and simultaneously decreases the time required to capture synaptogenic events by an order of magnitude. It is readily incorporated into multiwell formats compatible with industrial high-throughput screening platforms. Using this technology, we screened a chemical library, and identified novel histone deacetylase (HDAC) inhibitors that improve neuroligin-1-induced synaptogenesis by modulating class-I HDACs. We also found a structure–activity relationship for designing novel potent histone deacetylase inhibitors, which can be applied towards development of new therapeutics. Synapses are asymmetric intercellular junctions between neurons, which are crucial for transforming and transmitting signals [1] . Many abnormalities in brain function have direct or indirect effects on synaptic function or originate from synaptic dysfunction [2] , [3] , [4] , [5] , [6] . Hence, many therapeutic strategies for neurological diseases and disorders target synapses, and the development of high-throughput technologies for genetic and chemical screening of synaptic function is highly significant and necessary for both fundamental and therapeutic investigations. Synapse formation and plasticity involve successive and dynamic recruitment of pre- and postsynaptic molecules [7] , [8] , [9] . These processes are intricately regulated by the trans-synaptic adhesion proteins connecting pre- and postsynaptic terminals [10] , [11] , [12] . However, the bidirectional nature of synaptic signalling and the presence of a multitude of trans-synaptic signals make it complicated to separate direct effects from indirect effects on synapse assembly [13] , posing major challenges for the development of screening methods for many diseases where specific synaptic proteins are affected. Addition of purified synaptic adhesion proteins to primary neuron cultures is not suitable, because most synaptic adhesion proteins require membrane anchoring and lateral interactions to function normally [14] . To overcome these limitations, neuron–fibroblast cocultures have been employed, and have proven to be powerful tools for studying many aspects of synapse formation and function [15] . In these assays, primary neurons are cocultured with non-neuronal cells transfected with cDNA encoding only the specific synaptic proteins of interest. This provides significant control over the proteins involved in trans-synaptic signalling, and thus greatly reduces the complexity in dissecting the trans-synaptic signalling. Neuronal responses to the presented synaptic proteins can be measured using immunocytochemistry, fluorescence microscopy, image analysis tools, and electrophysiological approaches [16] . Such assays have been used to identify several adhesion proteins that modulate the synaptic function at pre- or postsynaptic terminals [15] , [17] , [18] , [19] , [20] , [21] , [22] . Among these synaptic adhesion proteins, neuroligins (NLGs) and neurexins (NRXs) are the most widely studied ones, and they have been shown to connect pre- and postsynaptic neurons, mediate signalling across synapses and modulate the properties of synaptic function. In humans, alterations in genes encoding NLGs or NRXs have recently been implicated in autism and other cognitive diseases [6] . Thus, coculture assays are promising tools for screens to discover synapse-organizing factors, and molecules or drugs that modulate synaptic function. However, existing coculture assays are not conducive to high-throughput screening for several reasons. Random distribution and occurrence of neuron–fibroblast and neuron-neuron interactions on culture substrates make it difficult to identify and analyse large and consistent numbers of synaptogenesis events. Fibroblast cells typically exhibit irregular morphologies or cluster together, severely hindering automated analysis. In addition, spatial variations in the density of randomly growing neurites on substrates create significant fluctuations in the quantification of synaptogenic events induced when neurites contact fibroblast cells, thereby reducing assay sensitivity. As a result, large numbers of cells are required in order to make statistically significant measurements, and subtle effects can be lost within experimental noise. Finally, densely packed neuronal somata near fibroblast cells may provide neurotrophic or other factors affecting synapse formation, and could indirectly bias the effects of presented synaptic proteins [23] . To overcome these challenges, we developed an unprecedentedly sensitive and scalable synapse assay technology that is also suitable for large-scale high-throughput screening purposes using both chemical and protein expression libraries. This synapse microarray technology overcomes the problems associated with the traditional coculture assays. It enables the induction of synaptic structures at pre-determined positions inside precisely controlled arrays of microwells, dramatically decreasing the time needed to capture synaptogenic events by approximately an order of magnitude, which is crucial for performing large-scale screens. Importantly, our technology also increases by tenfold the sensitivity of traditional coculture assays: we demonstrate that the synapse microarrays can detect synaptic changes induced by chemicals at tenfold lower concentrations. Such improvements in assay sensitivity, efficiency and repeatability are crucial for detection of subtle abnormalities in synaptic function, which are often associated with many severe brain disorders [3] , [4] , [5] , [6] . The platform also allows the use of minimal numbers of primary neurons and amounts of reagents in large-scale screens. Using this technology, we screened a chemical library at various concentrations. We identified novel histone deacetylase (HDAC) inhibitors that promote synapse formation through neuroligin-1 (NLG1). Many of these chemicals have subtle differential effects on synaptogenesis, which we quantified by using the synapse microarrays. Through analysis of the relationship between synaptogenic activity and the variations in chemical structures, we found a structure–activity relationship for designing novel potent HDAC inhibitors. In combination with a biochemical deacetylase assay using recombinant HDACs, we also showed that inhibition of class-I HDACs has an important role in NLG1-induced synaptogenesis. Design of the synapse microarray Previously, chemically patterned substrates [24] , [25] , soluble gradients [26] , physical structures that guide or compartmentalize neurites [27] , [28] have been employed to improve the organization of cultured neurons. Microfluidic platforms have also been used to conduct on-chip electrophysiology [29] , and to manipulate synaptic functions [30] . However, unlike the synapse microarrays introduced here, none of these techniques induces synapses in precise arrays for quantitative and high-throughput studies. The synapse microarrays consist of two main compartments connected by parallel microchannels (325 μm long, 10 μm wide and 3 μm high; Fig. 1 ), which have been previously shown to effectively isolate axons from neuronal somata [27] ( Supplementary Fig. S1 ). Dissociated neurons are plated and cultured in compartment 1 ( Fig. 1a ). The neural processes emanating from the somata grow through the microchannels and extend into compartment 2 ( Fig. 1b ), which is covered by a thin (80 μm) polydimethyl siloxane (PDMS) membrane held 3 μm above the substrate by small posts (10 μm diameter), which provide space for axonal outgrowth. The membrane also contains an array of through-holes (microwells with 30 μm diameter). After a dense axon network forms in compartment 2, HEK293 cells genetically engineered to express specific synapse-inducing transmembrane proteins are seeded into the microwells using a brief centrifugation. During rinsing, the cells captured within the holes are protected from shear stress, while the excess HEK293 cells are easily removed, leaving behind only the captured cells in the microwells ( Fig. 1c ). The resulting occupancy of the microarrays typically exceeds 90%, and over 85% of the microwells contain one to three HEK293 cells ( Supplementary Fig. S2 ). Cells are then cocultured for 1–2 days to allow for induction of synaptic structures. 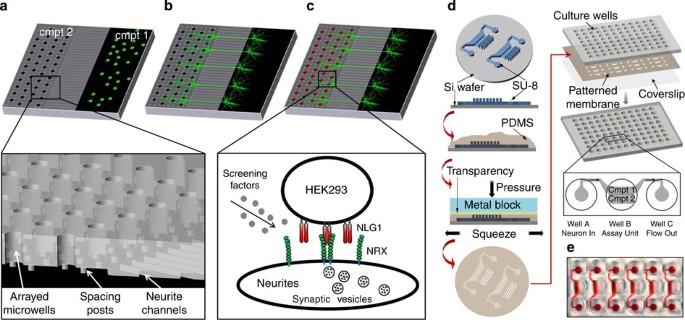Figure 1: Schematic of the synapse microarray technology. (a) Neuronal cells are loaded and cultured in compartment (cmpt) 1. (b) Neurites extend through the microchannels (325 μm long and 10 μm wide) and form a dense network in cmpt 2. Cmpt 2 is covered by a layer of 80-μm thick PDMS membrane containing 30-μm diameter through-holes (see inset in (a)). The membrane is held 3 μm above the substrate via dispersed 10-μm diameter posts (see inset in (a)). (c) HEK293 cells expressing NLG1 are then seeded into the through-holes, and cocultured with neurons for 1–2 days in the presence of screening factors before immunostaining for synaptic markers. In inset, NRX represents neurexin. (d) Fabrication of the synapse microarray. Polydimethylsiloxane (PDMS) prepolymer is poured onto a mould made from photoresist (SU-8) patterned on a silicon (Si) wafer. A plastic transparency is lowered onto the prepolymer. The mould/prepolymer/transparency stack is then clamped by two flat metal blocks, on which high pressure is applied to squeeze out extra prepolymer. A micropatterned PDMS membrane is released from the wafer after curing PDMS, and then sandwiched between a glass coverslip and multiwell-formatted culture wells to form the synapse microarrays. Each assay unit consists of three connected wells (also seeSupplementary Fig. S3). (e) A photograph of the synapse microarray in multiwell format. Figure 1: Schematic of the synapse microarray technology. ( a ) Neuronal cells are loaded and cultured in compartment (cmpt) 1. ( b ) Neurites extend through the microchannels (325 μm long and 10 μm wide) and form a dense network in cmpt 2. Cmpt 2 is covered by a layer of 80-μm thick PDMS membrane containing 30-μm diameter through-holes (see inset in ( a )). The membrane is held 3 μm above the substrate via dispersed 10-μm diameter posts (see inset in ( a )). ( c ) HEK293 cells expressing NLG1 are then seeded into the through-holes, and cocultured with neurons for 1–2 days in the presence of screening factors before immunostaining for synaptic markers. In inset, NRX represents neurexin. ( d ) Fabrication of the synapse microarray. Polydimethylsiloxane (PDMS) prepolymer is poured onto a mould made from photoresist (SU-8) patterned on a silicon (Si) wafer. A plastic transparency is lowered onto the prepolymer. The mould/prepolymer/transparency stack is then clamped by two flat metal blocks, on which high pressure is applied to squeeze out extra prepolymer. A micropatterned PDMS membrane is released from the wafer after curing PDMS, and then sandwiched between a glass coverslip and multiwell-formatted culture wells to form the synapse microarrays. Each assay unit consists of three connected wells (also see Supplementary Fig. S3 ). ( e ) A photograph of the synapse microarray in multiwell format. Full size image Synapse microarrays can be fabricated using conventional soft-lithography techniques as illustrated in Figure 1d . Large-scale screens require use of multiwell plates. Synapse microarrays are also easily adaptable to multiwell plate format because they do not require complex fluidic inputs and outputs. The micropatterned PDMS membrane is simply sandwiched between a standard glass coverslip and multiwell-formatted culture wells. Each 96-well plate can perform 32 complete assays, where each assay unit consists of three connected wells. First, neuronal cells are loaded into well A by direct pipetting. The neurons then passively flow into compartment 1 in well B, which is coated with cell adhesion proteins. After 7 days, HEK293 cells are pipetted and seeded into compartment 2 of well B as described above. Well C is used for liquid exchange ( Fig. 1d,e ; Supplementary Fig. S3 ). This design is also easily adaptable to 24-well, 48-well and 384-well format plates. Precise control of neuron–fibroblast cocultures The synaptogenic activity in coculture assays is assessed by the fluorescence measurements of the synaptic clustering colocalized with HEK293 cells. An initial step in the induction of these clusters is the formation of contacts between the axons and NLG1-expressing HEK293 cells, which depends both on neurite distribution and on spreading of HEK293 cells. As neurite density varies spatially, the number of synapses that form when neurites contact HEK293 cells fluctuate accordingly. We first examined whether our synapse microarray system improves the uniformity of neurite density within the microwell array. We measured the distribution of total neurite lengths in randomly sampled regions (30 μm in diameter) of a traditional coculture, and compared it with those measured in microwells of synapse microarrays ( Fig. 2 ). In traditional cultures, neurite density varies dramatically due to uneven growth of neurons ( Fig. 2a ). In particular, neurite density significantly depends on the distance from the soma due to neurite branching [31] , which is not controlled in traditional cultures. In the synapse microarrays, the somata are separated from HEK293 cells in microwells by a well-defined distance determined by the length of the microchannels. The resulting neurite density within the microwells is significantly more uniform as compared with traditional cultures ( Fig. 2c , P <0.01, n =3, analysis of variance (ANOVA) test, Fig. 2b versus d ). The coefficient of variation (CV) for neurite length distribution in the synapse microarray (0.24±0.02, mean±s.e.m.) is nearly half that of the traditional culture (0.47±0.04, mean±s.e.m.). HEK293 cells plated onto the microwell array therefore encounter a more uniform neurite distribution than they would do in a traditional coculture assay. 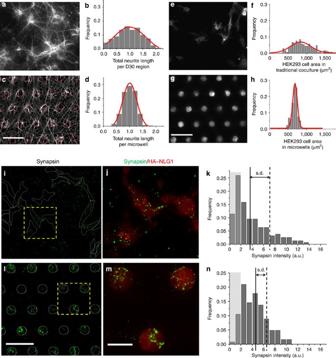Figure 2: Precise control of the neuron–fibroblast coculture by synapse microarrays. (a) A representative βIII-tubulin fluorescence image of neurites in traditionally dissociated neuron culture. (b) Distribution of total neurite length (normalized to mean) in randomly sampled regions of 30 μm diameter in a traditional culture (n=247). (c) βIII-tubulin fluorescence image of neurites in the synapse microarray. The microwells are circled in red, scale bar, 100 μm. (d) Distribution of total neurite length (normalized to mean) in microwells within 500 μm distance from the end of the microchannels guiding neurites (n=270). (e) HEK293 cells spread in varying morphologies in traditional cultures (staining for HA–NLG1). (f) Histogram of HEK293 cell area in traditional cultures (n=222). (g) HEK293 cells grow in well-defined morphologies in the synapse microarray (staining for HA–NLG1), scale bar, 100 μm. (h)Histogram of HEK293 cell area in the synapse microarray (n=286). (i) Fluorescence image of synapsin clustering associated with NLG1-transfected HEK293 cells (outlined in white) in traditional cocultures. (j) Enlarged view of the boxed region in panel (i) (synapsin, red; HA–NLG1, green). (k) Histogram showing the distribution of synapsin fluorescence intensity colocalized with HEK293 cells in traditional cocultures (n=160). (l) Fluorescence image of synapsin clustering in microwells (white circles) filled with HEK293 cells, scale bar, 100 μm. (m) Enlarged view of the boxed region in panel (l) (synapsin, red; HA–NLG1, green), scale bar, 30 μm. (n) Histogram showing the distribution of synapsin fluorescence intensity in microwells (n=248). In panels (k) and (n), light grey-covered columns indicate the proportion of regions with substantially low synapsin fluorescence. One standard deviation from the mean values (solid lines) is indicated by the dashed lines. Figure 2: Precise control of the neuron–fibroblast coculture by synapse microarrays. ( a ) A representative βIII-tubulin fluorescence image of neurites in traditionally dissociated neuron culture. ( b ) Distribution of total neurite length (normalized to mean) in randomly sampled regions of 30 μm diameter in a traditional culture ( n =247). ( c ) βIII-tubulin fluorescence image of neurites in the synapse microarray. The microwells are circled in red, scale bar, 100 μm. ( d ) Distribution of total neurite length (normalized to mean) in microwells within 500 μm distance from the end of the microchannels guiding neurites ( n =270). ( e ) HEK293 cells spread in varying morphologies in traditional cultures (staining for HA–NLG1). ( f ) Histogram of HEK293 cell area in traditional cultures ( n =222). ( g ) HEK293 cells grow in well-defined morphologies in the synapse microarray (staining for HA–NLG1), scale bar, 100 μm. ( h) Histogram of HEK293 cell area in the synapse microarray ( n =286). ( i ) Fluorescence image of synapsin clustering associated with NLG1-transfected HEK293 cells (outlined in white) in traditional cocultures. ( j ) Enlarged view of the boxed region in panel ( i ) (synapsin, red; HA–NLG1, green). ( k ) Histogram showing the distribution of synapsin fluorescence intensity colocalized with HEK293 cells in traditional cocultures ( n =160). ( l ) Fluorescence image of synapsin clustering in microwells (white circles) filled with HEK293 cells, scale bar, 100 μm. ( m ) Enlarged view of the boxed region in panel (l) (synapsin, red; HA–NLG1, green), scale bar, 30 μm. ( n ) Histogram showing the distribution of synapsin fluorescence intensity in microwells ( n =248). In panels ( k ) and ( n ), light grey-covered columns indicate the proportion of regions with substantially low synapsin fluorescence. One standard deviation from the mean values (solid lines) is indicated by the dashed lines. Full size image In addition, in traditional coculture assays, the spreading area of HEK293 cells shows significant variation (900±306 μm 2 , mean±s.d., Fig. 2e,f ), which affect the quantification of synaptic clusters formed on individual HEK293 cells ( Supplementary Fig. S4 ). Although the measurement of synaptic clustering can be normalized by the area of HEK293 cells, estimating the area of irregularly shaped HEK293 cells is often done manually and thus laborious. Hence, fluctuation in the area of HEK293 cells is another factor that leads to further variation in the estimate of synaptogenic activity. The synapse microarray overcomes this problem by confining the HEK293 cells within microwells. The synapse count does not show dependency on the number of HEK293 cells in microwells ( Supplementary Fig. S5 ), as the contact area between the neurites and HEK293 cells on the substrate is determined by the diameter of the microwells. The microwells both provide access for HEK293 cells to the uniform neurite network beneath the PDMS membrane and also constrain the growth and spread of HEK293 cells to a defined region (676±88 μm 2 , mean±s.d., Fig. 2g,h ). This confinement of HEK293 cells does not affect NLG1 protein expression levels ( Supplementary Fig. S6 ). To quantify presynaptic specialization induced by NLG1-expressing HEK293 cells, we immunostained for synapsin after coculturing HEK293 cells with dissociated neurons for 24‐–48 h ( Fig. 2i,j ). In traditional cocultures, we quantified synapses by measuring the total fluorescence of synapsin clusters within each manually outlined region covered by individual HEK293 cells. Figure 2k shows that synapsin clustering is quite heterogeneous (CV=0.89±0.08, mean±s.e.m. ), and is substantially weak ('inactive') for a large fraction (38±2%) of the HEK293 cells. In the microarray system, synapses were quantified by measuring the total synapsin fluorescence in each microwell. The synapse distribution in the microarray ( Fig. 2l,m ) was significantly more homogeneous (CV=0.55±0.06, P <0.01, one way ANOVA, n =3), as shown in Figure 2n . The inactive proportion of sampled regions was also significantly less than that of traditional cocultures (13±1%). Additionally, the distribution of synapsin puncta size is not affected by the synapse microarray in comparison with the traditional coculture method ( Supplementary Fig. S7 ). Sensitivity analysis of synapse microarray technology To demonstrate the capability of our synapse microarray technology for capturing synaptogenic events in the presence of exogenously added chemicals, we first quantified the effects of a known HDAC inhibitor on NLG1-induced presynaptic specialization. HDAC inhibitors have already been shown to facilitate the development and function of excitatory synapse in vitro [32] , and also to enhance memory-related behaviour in rodent models [33] , [34] , [35] . We found that the HDAC inhibitor, trichostatin A (TSA), significantly enhanced NLG1's ability to induce presynaptic clustering, as compared with non-treated samples ( P <0.001; Fig. 3a ). This enhancement was not due to changes in the NLG1 expression levels in HEK293 cells after TSA treatment ( Fig. 3b ). 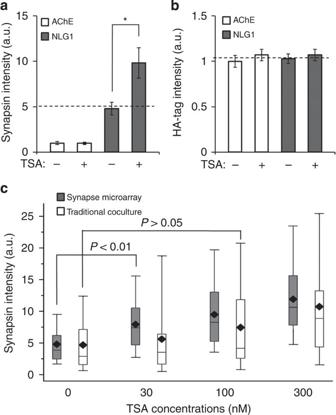Figure 3: Sensitivity analysis of the synapse microarray technology. (a) Effects of TSA on NLG1-induced synapsin clustering detected by synapse microarrays. *P<0.001 by ANOVA analysis. (b) Fluorescence intensities for HA–NLG1 or HA–AChE showing NLG1 expression levels in HEK293 cells under each condition examined. For panels (a,b), error bars indicate s.e.m. from four independent experiments. For each experiment, 200 microwells were analysed for each condition, and the fluorescence intensities were normalized to the control using AChE-transfected HEK293 cells. (c) Detection of TSA's effects on NLG1 induced presynaptic clustering as a function of TSA concentrations. Box plots of synapsin fluorescence intensities from assays using either the synapse microarray (grey columns) or traditional coculture (white columns). The whiskers and elements of the boxes correspond to 5, 25, 50, 75 and 95 percentiles of the data, whereas the diamond corresponds to the dataset mean. Each box contains differing numbers of events collected from equal number of images. Statistical significance was determined by Kruskal–Wallis analysis. Figure 3: Sensitivity analysis of the synapse microarray technology. ( a ) Effects of TSA on NLG1-induced synapsin clustering detected by synapse microarrays. * P <0.001 by ANOVA analysis. ( b ) Fluorescence intensities for HA–NLG1 or HA–AChE showing NLG1 expression levels in HEK293 cells under each condition examined. For panels ( a , b ), error bars indicate s.e.m. from four independent experiments. For each experiment, 200 microwells were analysed for each condition, and the fluorescence intensities were normalized to the control using AChE-transfected HEK293 cells. ( c ) Detection of TSA's effects on NLG1 induced presynaptic clustering as a function of TSA concentrations. Box plots of synapsin fluorescence intensities from assays using either the synapse microarray (grey columns) or traditional coculture (white columns). The whiskers and elements of the boxes correspond to 5, 25, 50, 75 and 95 percentiles of the data, whereas the diamond corresponds to the dataset mean. Each box contains differing numbers of events collected from equal number of images. Statistical significance was determined by Kruskal–Wallis analysis. Full size image To characterize the synapse microarray's sensitivity for detecting changes in synaptogenesis, we performed a dose–response assay to measure the effect of TSA on NLG1-induced presynaptic specialization, and we compared these results to those produced by traditional coculture assays ( Fig. 3c ). Although traditional coculture assays allow detection of TSA-enhanced presynaptic clustering at 300 nM ( P <0.001), it fails to detect any effect at lower concentrations (that is, for 30 nM and 100 nM, P >0.05). On the other hand, the data acquired using our synapse microarray consistently showed a linear dose–response to TSA, and we were able to detect a significant increase in NLG1-induced presynaptic clustering, even at the lowest TSA dose tested (30 nM, P <0.01), indicating almost tenfold improvement in sensitivity over traditional coculture assays. Automated image acquisition and processing for screens Image acquisition and analysis of traditional coculture assays are typically performed manually, which are both labour intensive and error prone, especially for large-scale screening of chemical or cDNA libraries of synaptic proteins [21] . The synapse microarray, however, is exceptionally conducive to automated imaging and analysis. We use a standard fluorescence microscope equipped with an automated stage to scan and acquire images from three fluorescent channels (corresponding to HA-NLG1, synapsin and βIII-tubulin). Composite images are then analysed using custom-made software that identified microwells filled with HEK293 cells, and recorded the fluorescence intensity profiles of the different channels for statistical analysis ( Supplementary Movie 1 ). Thus, our synapse microarrays enable full automation of both data acquisition and image analysis without any manual intervention or special equipment. Table 1 shows that our platform is faster approximately by an order of magnitude than the traditional coculture assay even when larger number of data points are acquired by our platform. Such speed-up is crucial for conducting large-scale screens (see Discussion section). Table 1 Comparison of approximate time needed to analyse one sample for assays using synapse microarray versus traditional coculture. Full size table Screening of chemical libraries using synapse microarrays Inhibitors of general HDACs have been shown to enhance synapse development and function [32] , [34] . Yet, little is known about the mechanism connecting specific HDACs and their involvement in neuroregenerative activities and synaptogenesis. Identification of which subclasses of HDACs are important for synaptic function and discovery of selective inhibitors of these specific HDACs is highly desirable for therapeutic purposes. Akhtar et al . [32] recently showed that HDAC1 and HDAC2 are key regulators of synaptogenesis. To investigate whether HDACs are the relevant target for the synaptogenic effect of TSA on NLG1-dependent signalling that we observed and also to identify novel HDAC inhibitors effective in promoting synapse formation, we next screened a library of both known and novel HDAC inhibitors ( Supplementary Table S1 ) comprising three additional chemotypes selected to provide information on the subclass of HDACs involved. The novel HDAC inhibitors were initially selected after performing in vitro biochemical deacetylase assays using recombinant HDACs ( Table 2 ), but their effects on synapse formation in primary neurons were unknown a priori . Using the synapse microarrays, a total of 22 compounds were screened in a blinded fashion at three concentrations (0.1, 1 and 10 μM) in duplicate ( Fig. 4a,b ). The chemicals we tested included SAHA, LBH-589 and scriptaid, all of which are known potent hydroxamic acid-based HDAC inhibitors that are similar to TSA and have IC 50 values <5 nM for class-I HDACs in our deacetylase assays ( Table 2 ). Consistent with the effects of TSA, all three of these HDAC inhibitors were also potent in our coculture assay. In contrast, neither of the two compounds, valproic acid and phenylbutyric acid, affected synaptogenesis at highest concentration (10 μM) tested, which is consistent with their weak inhibition towardsclass-I HDACs in the deacetylase assay (IC 50 > 40 μM) ( Fig. 4c ). Table 2 IC 50 value (nM) of compounds towards specific HDACs tested in this study. 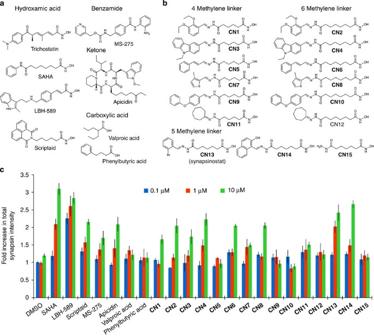Figure 4: Screening of known and novel HDAC inhibitors for small molecules modulating NLG1-induced synaptogenesis using synapse microarrays. (a) Four structural classes (hydroxamic acids, benzamides, ketones and carboxylic acids) of known HDAC inhibitors are tested. (b) Novel hydroxamic acid containing HDAC inhibitors with varying linker lengths and capping elements. (c) Fold increase in total synapsin intensity upon treatment of cultures with the indicated compounds at three different concentrations (0.1 μM, blue; 1 μM, red; and 10 μM, green). A compound is considered 'active' if it induces an at least 1.5-fold increase in total synapsin intensity over DMSO control level at tested concentrations. While a number of novel hydroxamic acid-containing compounds increased synaptogenesis at 10 μM concentration, onlyCN13(synapsinostat) is active at 1 μM. Full size table Figure 4: Screening of known and novel HDAC inhibitors for small molecules modulating NLG1-induced synaptogenesis using synapse microarrays. ( a ) Four structural classes (hydroxamic acids, benzamides, ketones and carboxylic acids) of known HDAC inhibitors are tested. ( b ) Novel hydroxamic acid containing HDAC inhibitors with varying linker lengths and capping elements. ( c ) Fold increase in total synapsin intensity upon treatment of cultures with the indicated compounds at three different concentrations (0.1 μM, blue; 1 μM, red; and 10 μM, green). A compound is considered 'active' if it induces an at least 1.5-fold increase in total synapsin intensity over DMSO control level at tested concentrations. While a number of novel hydroxamic acid-containing compounds increased synaptogenesis at 10 μM concentration, only CN13 (synapsinostat) is active at 1 μM. Full size image As these hydroxamates and TSA are known to inhibit both class-I and class-IIb HDACs [36] , [37] , we also tested non-hydroxamates that show improved selectivity for class-I HDACs (HDAC1/2/3/8). MS-275 is a benzamide class of HDAC inhibitor, which was moderately potent towards only the class-I HDAC1/2/3 in our deacetylase assay ( Table 2 ). This compound showed moderate potency in the coculture assay at the highest concentration tested (10 μM), causing ~1.5-fold increase in presynaptic clustering, compared with the DMSO control. To extend these results to another structural class of non-hydroxamates, we also tested apicidin, a natural product and one of the most potent class-I-selective HDAC inhibitors tested in our deacetylase assay ( Table 2 ). As expected, this compound showed greater potency than MS-275 in the coculture assay ( Fig. 4c ). Taken together, the results of MS-275 and apicidin suggest that the class-I HDACs have an important role in synaptogenesis induced by NLG1. To demonstrate the capability of our platform to identify novel molecules that can modulate synaptogenesis, we also included in the chemical library 15 novel HDAC inhibitors based upon hydrazone-coupling chemistry [38] . While all of these novel compounds showed strong inhibition of the class-I HDAC1-3 in our deacetylase assays ( Table 2 ), only some of them enhanced NLG1-induced synaptogenesis ( Fig. 4c ). Like TSA, these novel HDAC inhibitors all possess a hydroxamic acid, but have varying linker lengths and capping groups that differ from TSA ( Fig. 4a,b ). The capping group and linker region have been modified extensively towards the creation of class-selective or isoform-selective HDAC inhibitors [37] , [39] . For example, CN1 to CN2 differ by the number of the methylene groups in the linker region between the hydroxamate and hydrazone moieties: CN1 has a four methylene linker whereas CN2 has a six methylene linker. While both were potent HDAC inhibitors in the deacetylase assays, CN2 was more potent than CN1 ( Table 2 ). CN2 was also more potent than CN1 in the coculture assays ( Fig. 4c ), which correlates with its increased HDAC inhibitory potency over CN1 . A similar structure–activity relationship existed between other novel hydroxamate-containing compound pairs we have tested, containing four versus six methylene linkers (that is, CN3 and CN4 , CN5 and CN6 , and CN7 and CN8 ). In contrast to these correlations between the deacetylase assays and coculture assays, CN9 , CN10 , CN11 and CN12 were potent class-I HDAC inhibitors but none were active in the coculture assays. This indicates that in vitro biochemical assay on recombinant HDACs is necessary but not sufficient for observing an effect of compounds on synaptogenesis, highlighting the importance of cell-based assays for selecting useful modulators of HDAC-mediated processes. Of the novel compounds we screened, CN13 , here named synapsinostat, was found to be the most potent in promoting synaptogenesis, and it was effective even at the medium concentration (1 μM) tested. Synapsinostat ( CN13 ) contains only a 5-carbon methylene linker, similar to CN14 and CN15 . CN14 was also a strong inducer of synaptogenesis but only at higher concentrations (10 μM) while CN15 was inactive. CN14 and CN15 differ from synapsinostat ( CN13 ) by their capping elements. This demonstrates the importance of the capping element for synaptogenic activity of the hydroxamic acid-containing compounds. Taken together, screening a collection of HDAC inhibitors at different concentrations using synapse microarrays has provided insight for future synthetic chemistry efforts aiming to develop selective regulators of synaptogenesis. We have demonstrated an array-based coculture system for conducting synaptogenesis assays with unprecedented sensitivity and throughput over traditional assays. Synapse microarrays enable the induction of synaptic structures at pre-determined locations in regular arrays and eliminate several factors that cause experimental fluctuations in the traditional coculture assays. The high-throughput capability of the synapse microarray is crucial for conducting large-scale screens, allowing the acquisition and analysis of large amounts of data within a reasonable time scale. For example, performing a screen using traditional coculture assays involving a medium-size library of 100,000 chemicals would require several years if done with existing methods, while the time could be reduced to a few months if the screen is conducted using the synapse microarrays ( Table 1 ). Furthermore, the high sensitivity of the platform could enable the detection of subtle abnormalities in synaptic function associated with complex brain disorders [4] , [5] , [6] , which is a significant challenge for pharmaceutical screens. In addition, the higher sensitivity of synapse microarrays enables screening at significantly lower chemical concentrations, which is important for large-scale screens due to the substantial reagent costs, and because many compounds have off-target or toxic effects at higher doses [40] . The higher sensitivity and the small configuration of assays also allow use of minimal numbers of primary neurons, which are otherwise hard to obtain. Using this synapse microarray technology, we screened a chemical library of novel HDAC inhibitors, and identified chemicals, including synapsinostat ( CN13 ), that promote synapse formation through NLG1. Many chemicals have subtle differential effects on synaptogenesis, which we quantified by using synapse microarrays. Through analysis of the relationship between synaptogenic activity and the chemical structures, we found a structure–activity relationship for designing potent hydroxamate-containing HDAC inhibitors. We showed that the length of the methylene linker between the metal chelating moiety of the hydroxamic acid and capping element that extends towards the surface of the binding pocket has a key role in synaptogenic activity. In combination with in vitro biochemical deacetylase assays using recombinant HDACs, we also found that inhibition of class-I HDACs has an important role in the process of NLG1-induced synaptogenesis. These results are consistent with the previous findings of Akhtar et al . [32] , and further extend their findings by demonstrating that NLG1 is involved in mediating the effects of class-I HDAC inhibitors. There is accumulating evidence that HDACs inhibitors exhibit neuroprotective and neuroregenerative properties in cell culture and in animal models of various brain diseases [41] . Treatment with various HDAC inhibitors has emerged as a promising new strategy for intervention in neurodegenerative diseases. However, most of the HDAC inhibitors that have been tested in the context of neurological diseases are pan-HDAC inhibitors, that is, targeting HDACs non-selectively [42] . Prolonged broad-spectrum HDAC inhibition using such pan-HDAC inhibitors can be problematic, because these inhibitors have been associated with adverse side effects [43] , and different HDACs likely serve distinct regulatory functions within the adult brain [42] , [44] . Hence, screening and discovery of novel HDAC inhibitors is important for potential therapeutic applications, which can be achieved using the synapse microarray technology. With appropriate staining to subtype-specific synaptic markers (for example, vGlut1 and GAD65), the synapse microarray can be used to monitor differential effects of the small molecules on excitatory versus inhibitory synapses ( Supplementary Fig. S8 ). While the assays in our study targeted the NLG1 pathway, other synaptic proteins aside from NLG1 can also be used in chemical or RNAi screens. Similarly, using pools of HEK293 cells that are transected with cDNA encoding different synaptic proteins, the synapse microarrays can also be used to screen a library of candidate synapse-inducing proteins, as recently demonstrated by Linhoff et al . [21] using traditional cocultures. With little modification, the synapse microarrays can be easily adapted to study dendritic and postsynaptic development ( Supplementary Fig. S9 ), as well as to study various interactions among subtypes of neurons, or between neurons and other types of cells in the nervous system, such as astrocytes and oligodendrocytes. Synapse microarray fabrication The synapse microarray was made by assembling a standard coverslip, a micropatterned PDMS membrane and multiwell-formatted culture wells. The PDMS membrane was replica moulded from moulds fabricated by soft lithography [45] . The moulds consisted of three permanent SU-8 (Microchem) layers on a 4-inch silicon wafer. The first layer of SU-8 (3 μm in height) contained negative features for the supporting posts (in compartment 2) and the microchannels for neurite growth. The second layer of SU-8 (40 μm in height) contained negative features for the culturing channel in compartment 1. The third layer of SU-8 (80 μm in height) contained negative features for the microwells in compartment 2. All three layers were patterned sequentially by photolithography using a 20,000 dpi-printed transparency mask (CAD Art Services, Inc.). To create the micropatterned PDMS membrane, PDMS prepolymer was poured onto the mould and a plastic transparency was then carefully lowered onto the prepolymer. The mould/prepolymer/transparency stack was then clamped by two flat metal (aluminium) plates, on which high pressure was applied to squeeze out extra prepolymer [46] . The whole setup was baked at 85 °C for 12 h before releasing the patterned PDMS membrane (80 μm thick) from the mould. Cell culture Hippocampal neuron cultures were prepared following the method previously described [47] . Briefly, dissociated neurons were prepared from hippocampi dissected from E18 Sprague Dawley rats (Charles River) by enzymatic treatment with papain (Sigma) for 30 min at 37 °C followed by trituration with a 1 ml pipette tip. Before seeding neurons, all substrates were pre-coated with polylysine (Sigma, 100 μg ml −1 ) and laminin (Invitrogen, 10 μg ml −1 ). To characterize the synapse microarrays, we set up traditional and synapse microarray assays side by side, and compared them quantitatively. For the traditional neuron–fibroblast coculture assays, neurons were seeded onto 12-mm diameter coverslips at a density of 5×10 4 cm −2 . For assays using the synapse microarrays, 10 μl of the cell solution (at a cell density of 3×10 6 ml −1 ) was added to the cell-loading wells to achieve a cell density similar to that on the coverslips. This density yielded a uniform distribution of neurons in compartment 1. Neuron cultures were maintained in Neurobasal medium (Invitrogen) supplemented with B27, 0.5 mM L -glutamine and antibiotics for 7 days before coculture with HEK293 cells. Half the medium was replaced every 3–4 days. The coculture of HEK293 cells and neurons were performed essentially as previously described [16] . HEK293 cells were cultured according to standard procedures. The N-terminal HA-tagged murine NLG1 construct and the negative control construct, HA-tagged acetylcholinesterase (AChE), were generous gifts from Prof. Peter Scheiffele. HEK293 cells were transfected with the constructs using Lipofectamine (Invitrogen), and maintained in Dulbecco's modified Eagle's medium medium containing 10% foetal bovine serum and geneticin (G418, Invitrogen). The transfected cells were trypsinized and collected as a cell suspension (1×10 5 ml −1 ). For traditional coculture assays, HEK293 cells were seeded at a density of 2×10 4 cm −2 . For assays using synapse microarrays, 100 μl of the HEK293 cell suspension was added to each assay unit. The plate was centrifuged briefly at 100 g to allow the HEK293 cells to settle into the microwells, and extra cells were rinsed away via medium exchange. The cocultures were maintained in neurobasal medium for 24–48 h with addition of appropriate chemicals at various concentrations. In all assays, chemicals were added to both cell body and axon compartments of the synapse microarrays. Immunocytochemistry For analysis, cocultures were fixed for 30 min in 4% paraformaldehyde in phosphate-buffered saline (PBS), permeablized in 0.25% Triton X-100 for 20 min and then blocked with 4% bovine serum albumin in PBS for 2 h at room temperature or overnight at 4 °C. Cultures were incubated with primary antibodies in 4% bovine serum albumin for 2 h at room temperature, rinsed with PBS, incubated with secondary antibodies for 1 h and were again rinsed with PBS before imaging. Primary antibodies included chicken anti-HA (Millipore), rabbit anti-synapsin (Millipore), mouse anti-βIII-tubulin (R&D), mouse anti-Tau1 (Millipore), rabbit anti-MAP2 (Millipore), mouse anti-vGlut1 (Millipore) and rabbit anti-GAD65 (Millipore). Image acquisition and quantification Stained samples were imaged on a Nikon Eclipse TE2000 microscope (Nikon) equipped with a motorized stage, cooled CCD camera and a ×20 objective (0.75 numerical aperture). For quantification, all samples within one experiment were stained simultaneously and imaged with identical settings. For assays using the synapse microarrays, 10–15 images of the microwell area were taken within 500 μm distance from the microchannels guiding neurites. For traditional coculture assays, 10–15 images were taken at random positions on the substrate. All imaging and analysis were performed blindly to the synapsin channel. To quantify synapsin fluorescence, all synapsin fluorescent images within one experiment were thresholded equally. For the traditional coculture assays, contours of the transfected HEK293 cells (visualized by the HA–NLG1 fluorescent images) were manually outlined and chosen as the regions of interest (ROIs). For assays using synapse microarrays, the microwells filled with HEK293 cells were automatically selected as ROIs. Fluorescence intensity in ROIs for both synapsin and HA tag were quantified and normalized to the negative control using AChE-transfected HEK293 cells included in each experiment. The analysis procedures for assays using synapse microarrays were automated using a custom Matlab script. To quantify the total neurite length within each microwell (for assays using microarrays) or within randomly sampled 30 μm diameter regions (for traditional coculture assays), the βIII-tubulin fluorescence images were thresholded equally, and then skeletonized for measurement of total neurite length, which was further normalized to the mean value in order to visualize and quantify the dispersion and the distribution of the data. Screening of compounds affecting synaptogenesis TSA, SAHA, LBH-589, scriptaid, MS-275, apicidin valproic acid and phenylbutyric acid were purchased from commercial vendors. All novel compounds ( CN1 -15) were made following our published protocol [48] . The purity of the novel compounds was determined by analytical liquid chromatopgraphy–mass spectrometry using a Waters 2545 HPLC equipped with a 2998 diode array detector, a Waters 3100 eESI-MS module, using a XTerraMS C18 5 μm, 4.6×50 mm HPLC column at a flow rate of 5 ml min −1 with a linear gradient (95% A: 5% B to 100% B 90 s and 30 s hold at 100% B, solvent A=water+0.1% formic acid, solvent B=acetonitrile+0.1% formic acid, see Supplementary Fig. S10 ). Compounds were added to the synapse microarray by replacing culture medium containing appropriate concentrations of each compound. A compound is considered 'active' if it induces an at least 1.5-fold increase in total synapsin intensity over DMSO control level at tested concentrations (0.1, 1 and 10 μM). HDAC biochemical deacetylase assays Recombinant HDAC1, HDAC2, HDAC3, HDAC5, HDAC6 and HDAC8 were purchased from BPS Biosciences. Assays of recombinant HDAC deacetylase activity were performed with class-specific synthetic peptide substrates as described by Bradner et al . [36] How to cite this article: Shi, P. et al . Synapse microarray identification of small molecules that enhance synaptogenesis. Nat. Commun. 2:510 doi: 10.1038/ncomms1518 (2011).